Self-assembling knots of controlled topology by designing the geometry of patchy templates The self-assembly of objects with a set of desired properties is a major goal of material science and physics. A particularly challenging problem is that of self-assembling structures with a target topology. Here we show by computer simulation that one may design the geometry of string-like rigid patchy templates to promote their efficient and reproducible self-assembly into a selected repertoire of non-planar closed folds including several knots. In particular, by controlling the template geometry, we can direct the assembly process so as to strongly favour the formation of constructs tied in trefoil or pentafoil, or even of more exotic torus knots. Polydisperse and racemic mixtures of helical fragments of variable composition add further tunability in the topological self-assembly we discovered. Our results should be relevant to the design of new ways to synthesize molecular knots, which may prove, for instance, to be efficient cargo-carriers due to their mechanical stability. Self-assembly, at multiple length scales, is an important goal of material science and of physics, and recent times have witnessed a marked rise in research efforts aimed at discovering new ways in which this objective may be achieved. For instance, colloidal scientists and soft matter physicists have explored the feasibility of self-assemblying extended photonic crystals and other metamaterials by designing patchy particles of increasingly complex surface activity [1] , [2] , [3] , [4] , by exploiting the shape anisotropy of convex polyhedrical colloids [5] , [6] or by choosing to disperse particles into complex fluids such as binary fluids or liquid crystals [7] , [8] , [9] , [10] . The resulting interparticle interactions are in general highly non-trivial and can promote the formation of crystals, glasses, gels and so on, often with tunable physical properties [11] . In other cases, the goal of self-assembly is the formation of a target structure, at a length scale only slightly larger than that of the microscopic constituents. A beautiful example is provided by the creation of DNA origami [12] , [13] , [14] , or of other DNA-based microstructures, such as molecular spiders and nanorobots [15] , [16] , [17] . Here various target structures can be achieved by favouring the base pairing of specific DNA regions, which embody the struts of the desired construct. The DNA assembly technology is nowadays so advanced that planar structures can be designed in fully automated processes [18] . Here we address a related, yet distinct, problem: we wish to design string-like rigid templates that can spontaneously assemble in solution to form fully three-dimensional (3D) closed structures with a specified topology. Unlike previous seminal work that considered clusters of dipolar spheres [19] , or flexible colloidal and biological polymers with tunable chemical interactions [20] , [21] , in our framework knots are created starting from a variable number of identical rigid monomeric fragments, which join up thanks to simple, non-specific attractive interactions. This simplicity is a notable advantage in view of future experimental realizations of our in silico self-assembly. Accordingly, we shall exclusively vary the shape of the templates and ask whether this suffices to design a set of conditions under which the templates spontaneously self-assemble into, say, a trefoil knot or another prescribed knot type. This problem of the self-assembly of target topologies (henceforth ‘topological self-assembly’) with string-like fragments is important from a fundamental point of view. In fact, the thermodynamic and kinematic pathway to tie a polymer chain into a given 3D molecular knot is intricate and extremely challenging to incorporate in a self-assembly protocol [20] ; this matter is at the basis of the known difficulty of naturally occurring knotted proteins to fold without the aid of molecular chaperones [22] . Gaining a better understanding of this problem may be useful in practical contexts too; for example, to harness the mechanical stability of knotted structures to engineer better molecular cages for nanoreactors, or other cargo-carrier constructs. It may further provide a route to design novel synthetic molecular knots, if templates of small enough size can be fabricated. This would extend the current range of synthetic molecular topologies which, notwithstanding recent major technical advancements [23] , [24] , [25] , [26] , [27] , [28] , is still presently limited. Towards these goals we consider monodispersed solutions of helical building blocks with sticky (patchy) ends and show that it is possible to optimally design their geometry so to favour the spontaneous and efficient self-assembly into closed constructs with different topologies. In particular, we found that the most robustly designable knot types are two torus knots: the trefoil knot and the 8 19 knot. The latter has apparently not yet been considered in molecular architecture contexts and hence is an ideal candidate for future experimental attempts. Finally, we show that the repertoire of designable topologies can be significantly extended by considering solutions where helical templates of different shape or chirality are mixed. Protocol As the basic shape for the self-assembling templates we considered helical fragments. On one hand, this is because, their curved shape and non-planar nature are naturally compatible with the properties of closed 3D structures, including the knotted ones that we wish to assemble. On the other hand, helices can be analysed quite simply mathematically, as the whole repertoire of inequivalent shapes of their centre line is spanned by two parameters only: the projected opening angle, α and the longitudinal span or height, h , normalized to the radius of the circular projection, see Fig. 1a . 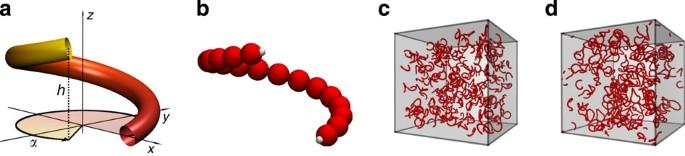Figure 1: Assembly templates and simulation setup. (a) The template centre line follows a helical curve projecting a unit radius and has angular and axial spans equal toαandh, respectively. Its Cartesian parametrization is {cos(αu), sin(αu),hu} withu∈[0,1]. (b) The helical centre line is next threaded with spherical beads of diameterσ=1/3 (red spheres,σis in units of the projected helical radius, as all other distances) and its termini are functionalized with small attractive patches (white spheres). (c) Initial configuration of 250 identical rigid templates (α=1.7πandh=1.6) packed inside a periodic simulation box at a volume fraction of about 0.56%. The templates interact exclusively via their excluded volume repulsion and the short-ranged attraction of the patches. The spontaneous assembly kinetics of the templates is followed by integrating numerically the Langevin dynamics of the system. A typical system configuration at steady state is shown in panel (d). Figure 1: Assembly templates and simulation setup. ( a ) The template centre line follows a helical curve projecting a unit radius and has angular and axial spans equal to α and h , respectively. Its Cartesian parametrization is {cos( αu ), sin( αu ), hu } with u ∈ [0,1]. ( b ) The helical centre line is next threaded with spherical beads of diameter σ =1/3 (red spheres, σ is in units of the projected helical radius, as all other distances) and its termini are functionalized with small attractive patches (white spheres). ( c ) Initial configuration of 250 identical rigid templates ( α =1.7 π and h =1.6) packed inside a periodic simulation box at a volume fraction of about 0.56%. The templates interact exclusively via their excluded volume repulsion and the short-ranged attraction of the patches. The spontaneous assembly kinetics of the templates is followed by integrating numerically the Langevin dynamics of the system. A typical system configuration at steady state is shown in panel ( d ). Full size image The building blocks used in our simulations are obtained by threading the centre lines of these helical fragments with identical spherical particles of diameter σ =1/3 (again, in units of the projected helical radius) interacting via a short-ranged repulsive Weeks–Chandler–Andersen potential. To make the templates stick to one another, the templates’ termini are functionalized with the same type of cohesive patch ( Fig. 1b ). The attractive interpatch interaction is modelled by a Gaussian potential with a strength of 25 k B T and interaction range of 0.1 σ . These parameters ensure two important properties. First, they guarantee that the bonding of contacting fragments is long lived. In fact, their typical pairwise unbinding time exceeds by several orders of magnitude the template Brownian time, that is, the time that a template needs to diffuse its own size under conditions of infinite dilution. Second, they ensure that the bonding can be established for a wide range of contact angles (see Supplementary Fig. 1 ). More details on the potential and simulation algorithms are given in the Methods section. We typically considered suspensions of 250 monodisperse right-handed helical fragments, inside a periodic cubic simulation box at a φ =0.56 % volume packing fraction. These parameters are chosen as typical of self-assembly in the dilute regime because they lead to an interfragment distance is comparable to the size of each fragment (see Methods). Starting from a random, non-overlapping initial arrangement of the templates, see Fig. 1c , the system dynamics is followed for a time span which is ∼ 500-fold longer than the time required by one template to diffuse over distances comparable to the initial mean separation of the templates. Over such time scales, the number of freely diffusing monomeric helical fragments gets depleted as templates bind to each other, and eventually reaches a limiting concentration, see Methods. At steady state, there is also a distribution of oligomeric chains, some of which are closed (circularized) while others are linear and hence open. Branched constructs, while theoretically possible, are disallowed by our choice of a suitably small interaction range between the ends of the templates (see Methods for details). 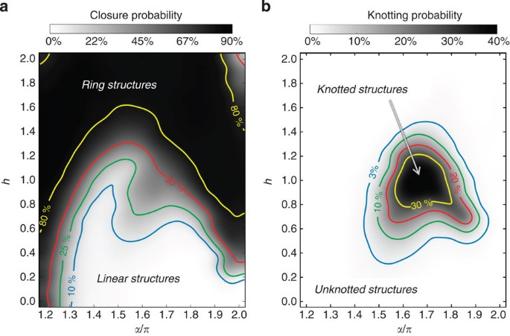Figure 2: Closure and knotting probabilities of the assembled constructs as a function of the templates shape parameters. The quantities shown inaandbare the closure and knotting probabilities of the self-assembled constructs. These probabilities are more rigorously defined in our framework as the percentage of templates involved in closed (a) and knotted (b) constructs, respectively. The phase diagram is drawn by interpolating data obtained by sampling the two-dimensional parameter space with a triangular grid withα/πandhspacings both equal to 0.1.his measured in units of the projected helical radius. Closure and knotting probability Figure 2a portrays how the fraction of templates in closed rings, also known as the closure probability, depends on the h and α parameters, which determine the shape of the template. The data show that relatively small variations in the geometry of the helical building blocks lead to sharp changes in closure probability: it is this extreme sensitivity that will make our topological self-assembly highly tunable. Figure 2: Closure and knotting probabilities of the assembled constructs as a function of the templates shape parameters. The quantities shown in a and b are the closure and knotting probabilities of the self-assembled constructs. These probabilities are more rigorously defined in our framework as the percentage of templates involved in closed ( a ) and knotted ( b ) constructs, respectively. The phase diagram is drawn by interpolating data obtained by sampling the two-dimensional parameter space with a triangular grid with α / π and h spacings both equal to 0.1. h is measured in units of the projected helical radius. Full size image A simple example that illustrates this behaviour is provided by the case for h =0, which corresponds to planar arcs. Figure 2a shows that, in the size range that we consider, these arcs are very unlikely to form closed loops, as the closure probability is close to zero. There is however an exception: if the template is approximately half a ring ( α ∼ π ), then dimerization leads to a perfect circle—correspondingly, there is a major rise in the closure probability, which approaches 1. In general, the sensitive dependence of the self-assembly output on the template geometry reflects two fundamental principles of configurational selection, one based on excluded volume and entropic constraints, the other on topological ones. Entropic considerations are particularly important to determine binding probability between templates: for certain template shapes it may even be sterically impossible for these to bind to each other; this happens, for instance, in the right corner region in Fig. 2a , see also Supplementary Fig. 2 . More generally, simple geometrical considerations clarify that excluded volume effects also preclude the formation of three-fragment rings (the most abundant component of closed structures in our simulations) in about one-third of the whole-phase space, see Supplementary Fig. 2 . On top of this, the incidence of closed conformations is further hindered by the decrease in entropy associated with oligomerization and binding. Given these premises, it is even more remarkable that, in broad regions of the parameter space, the incidence of self-assembled rings, including dimeric ones, can exceed 80% ( Fig. 2a ). Topological constraints also have a role: most notably, all ring-like structures may be characterized by their ‘total curvature’, which is simply the integral of the local radius of curvature over the ring length. The self-assembly of closed loops with a non-trivial knot topology, which are of particular relevance for our work, requires that the total curvature of the ring must be equal or exceed 4 π , and this leads to further selection in parameter space [29] as it poses a lower bound to the number of templates required for assembly. Having characterized the probability of forming circular structures, we next profiled their topology and found, remarkably, that many of these structures are knotted. Intriguingly, knots are most likely for non-planar templates located at the boundary between open and closed structures, see Fig. 2b . In fact, at the centre of the approximately convex region of phase space shown in Fig. 2b , as many as 50% of the 250 fragments are involved in knotted constructs. Observed knots repertoire The repertoire of knots which self-assemble in silico is impressively rich given the simplicity of the template shapes considered here, and is shown in Fig. 3a,b . All the observed knots are chiral (for example, the amphichiral Flemish knot 4 1 is not observed) and, unsurprisingly their chirality matches that of the templates used in the self-assembly. Moreover most of the knots are torus knots (which can be drawn on the surface of a torus) while twist knots as the 5 2 knot are extremely rare. Among the torus knots, however, only the conformations of the 3-mer trefoil knot (3 1 ), of the 4-mer 8 19 knot and of the 5-mer 10 124 knot resemble the ideal shape of these knots, that is the configuration which minimizes the rope length used to tie them [30] , [31] . Furthermore, presumably because the range of allowed contact angles is fairly wide, several alternative closed constructs geometries and topologies can self-assemble from the same helical fragments. For instance, for h =0.8 and α =1.8 π one has knots of type 5 1 , 8 19 and 3 1 (the latter made with both 3 and 4 templates). 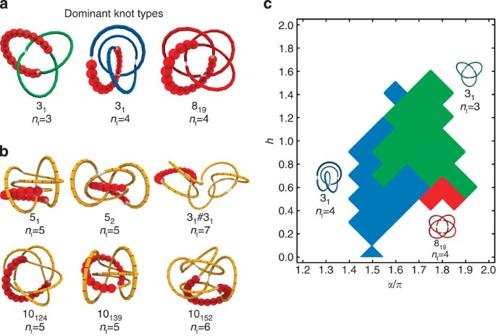Figure 3: Self-assembled knotted structures and topological phase diagram. (a) Representative conformers of the dominant self-assembled knots and (b) of other, rarer knot types. For visual clarity, only one of thentconstitutive templates is represented explicitly while for the others only the centre line is shown. The templates connecting regions are highlighted with white bonds. (c) Dependence of the dominant topology on the template geometry. In each coloured region the indicated knot is the dominant one, i.e. the non-trivial knot whose occurrence probability is highest and, in any case, not smaller than 1%. Following the left-to-right order shown in panel (a), the peak probability of the three dominant knot types is about 36, 12 and 3%, respectively.his measured in units of the projected helical radius. Figure 3: Self-assembled knotted structures and topological phase diagram. ( a ) Representative conformers of the dominant self-assembled knots and ( b ) of other, rarer knot types. For visual clarity, only one of the n t constitutive templates is represented explicitly while for the others only the centre line is shown. The templates connecting regions are highlighted with white bonds. ( c ) Dependence of the dominant topology on the template geometry. In each coloured region the indicated knot is the dominant one, i.e. the non-trivial knot whose occurrence probability is highest and, in any case, not smaller than 1%. Following the left-to-right order shown in panel ( a ), the peak probability of the three dominant knot types is about 36, 12 and 3%, respectively. h is measured in units of the projected helical radius. Full size image Dominant and robust knot types To gain more insight into our results, we present in Fig. 3c a topological ‘phase diagram’ showing the dominant type of knot—this is defined as the most frequent non-trivial knot which forms for a given choice of the h and α parameters. To avoid showing marginal or sporadic structures, in Fig. 3c we only consider knot types which appear with probability >1%. This topological phase diagram demonstrates that, by a suitable choice of the templates shape, it is possible to reliably control the statistical or thermodynamic incidence of self-assembled constructs with definite topology in a manner that is robust on decreasing or increasing the solution density by a factor of two, see Fig. 4 . Increasing the density ever further, for example, by a factor of 10, favours the formation of linear or percolating structures, at the expense of closed oligomeric constructs. Quite remarkably, however, within the observed dominant topologies for closed oligomers, which are shown in Fig. 4 , are identical to those previously discussed, see Fig. 3 . A further notable point is that closed constructs not only come in few distinct topologies, but are also locked into well-defined geometries. This geometrical monodispersity of the knotted assemblies is illustrated in Supplementary Fig. 3 . 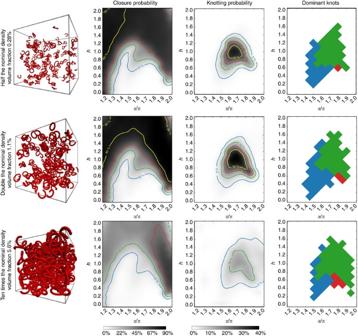Figure 4: Closure and knotting properties are robust against variation of templates concentration. The columns, from left to right, show snapshots, closure probability, knotting probability and topological phase diagrams. Results are obtained by packing the 250 templates to a monomer density that is half (first row), twice (second row) and 10 times (last row) as large as the reference one considered inFigs 1d,2a,band3c. The highest density favours the occurrence of constructs that are string-like or which percolate through the whole-simulation box. The occurrence of these structures reflects in a lower incidence of ring-like constructs. The high solution density can favour their linking; however, in the region of interest where the knotting probability is >5%, one observes that knotted rings take part in generic links in <6% of the cases. The topological phase diagram (dominant knots) is visibly robust throughout the wide range of densities studied. Figure 4: Closure and knotting properties are robust against variation of templates concentration. The columns, from left to right, show snapshots, closure probability, knotting probability and topological phase diagrams. Results are obtained by packing the 250 templates to a monomer density that is half (first row), twice (second row) and 10 times (last row) as large as the reference one considered in Figs 1d , 2a,b and 3c . The highest density favours the occurrence of constructs that are string-like or which percolate through the whole-simulation box. The occurrence of these structures reflects in a lower incidence of ring-like constructs. The high solution density can favour their linking; however, in the region of interest where the knotting probability is >5%, one observes that knotted rings take part in generic links in <6% of the cases. The topological phase diagram (dominant knots) is visibly robust throughout the wide range of densities studied. Full size image The topological phase diagram in Fig. 3c demonstrates that, of all knots that can be seen in simulations (shown in Fig. 3a,b ), those that are most abundant are only few. As shown in Fig. 3a , the dominant structures involve only two types of torus knots: trefoils, which occur in two geometrical flavours with 3 and 4 templates, respectively, and 8 19 knots. In knot tables, the 8 19 is marked as the first non-trivial torus knots because, if cut open, it presents three braided strands rather than two as the simpler 3 1 , 5 1 and 7 1 torus knots. It is remarkable that such a complicated knot as 8 19 has a much higher incidence than the 5 1 and 7 1 torus knots, which could be expected to be frequently assembled from chiral templates given their nominal simplicity (and which, in fact, are entropically favoured in fluctuating polymer chains [32] , [33] ). Importantly, the 8 19 knot and most of those shown in Fig. 3 —namely 3 1 , 5 1 , 10 124 and 10 139 knots—are also among the very few topologies that clusters of dipolar spheres can adopt to minimize their potential energy [19] . The unexpectedly broad overlap of the topologies that are viable for both our helical fragments and for chiral string-like clusters of dipolar spheres has, we believe, important implications. It suggests that these knots have various characteristics (chirality, compactness, symmetry and uniformity of curvature), which favour them markedly over other structures, as products of a thermodynamical self-assembly based on rather simple interactions. At the same time, it is interesting to note that, instead, the set of knots in Fig. 3 do not resemble the repertoire of topologies commonly formed by biopolymers such as proteins and DNA, whether in solution or under confinement [34] , [35] , [36] , [37] , [38] , [39] , [40] , [41] . Arguably, a key element favouring the self-assembly of the knots in Fig. 3a in our system is the chirality and intrinsic curvature of the building blocks. Consistent with this view, when repeating the self-assembly simulations for straight, rather than helical, fragments, we observed that the knotting probability dropped to negligible levels, see Supplementary Fig. 4 . Knots repertoire expansion by polydispersed templates The results presented thus far have been obtained using monodisperse template suspensions. What about mixtures, or polydisperse suspensions? To address this issue, we consider a situation in which a fraction x of the templates have a shape that promotes 3-template trefoils ( α =1.7 and h =1.0), whereas the remaining 1− x fraction has a geometry which directs the self-assembly of 8 19 knots, see Fig. 5 . A notable outcome of this numerical experiment is that the transition from the trefoil-dominated to a 8 19 -dominated regime is accompanied by the non-monotonic occurrence of the pentafoil 5 1 -knot type, which is virtually absent in either of the two pure phases. This suggests that the mixing ratio, x , provides a further dimension in the topological phase diagram of Fig. 3c , which can not only move around the boundary between different dominant knot types, but also introduce new structures, not observed for monodisperse suspensions. 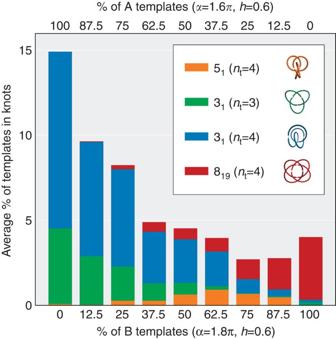Figure 5: The type and abundance of knots can be modulated in binary mixtures of templates. Throughout the explored mixing range, the overall volume fraction occupied by the 250 bi-dispersed templates was kept constant and equal to 0.56%.his measured in units of the projected helical radius. Figure 5: The type and abundance of knots can be modulated in binary mixtures of templates. Throughout the explored mixing range, the overall volume fraction occupied by the 250 bi-dispersed templates was kept constant and equal to 0.56%. h is measured in units of the projected helical radius. Full size image Another possible bidisperse suspension is a racemic mixture where the templates making up the two components are mirror images (that is, they have the same value of h but opposite values of α , one is right handed and the other one is left handed). This case also affects the outcome of our topological self-assembly, as racemic mixtures result in a marked decrease in the closure probability, and also in knot formation, see Supplementary Fig. 5 . It is also intriguing that achiral knots, which are not observed in monodisperse suspensions of templates with the same handedness, remain absent in these globally achiral racemic mixture. In conclusion, we have shown here that rigid helical templates with functionalized, sticky ends can be properly designed to self-assemble into a wide range of non-trivial topological structures, including a variety of torus knots, and some rare twist knots. Importantly, we have shown that in a dilute monodisperse suspension, there is a large region of parameter space where closed structures are more likely than open ones. Within this region we can further tune the parameters describing the basic geometry of the template to control efficiently and in a reproducible manner the knot type that is statistically dominant. Such dominant topologies can be the unknot, the trefoil knot as well as the more exotic 8 19 torus knot, one of the so-called Pretzel knots, which has eight crossings in its minimal projection and is known to topologists mainly because it provides the simplest example of a non-alternating torus knot [42] . Considering, instead, suspensions of polydispersed helical templates leads to further surprises. For instance by mixing templates which favour the formation of trefoils and 8 19 knots, respectively, we find that pentafoil knots, practically absent in the monodisperse topological phase diagram, can now be observed. Another interesting avenue in which our work can be further pursued in the future could be to allow to for some flexibility of the templates, as would be relevant for molecular or polymeric building blocks [26] . Designing molecular knots Our topological self-assembly is an example of thermodynamic self-assembly, or ‘passive’ self-assembly in the terminology of ref. 43 . Normally, we are used to the idea that thermodynamics can only drive the formation of relatively simple structures, whereas further information, or coding, is required to form more complicated assemblies which are often found in the living world. Against this conventional framework, our topological self-assembly provides a notable counter example: while lacking any active coding and while working in the absence of any external energy input, it can be tailored to drive the formation of knotted structures, with relatively high probability. It is especially remarkable that the selected knots are not in general the simplest ones, as we are able to self-assemble an 8-crossing knot as well as the trefoil and pentafoil knots. It would be of high interest to recreate our in silico topological self-assembly at the molecular level. At a mesoscopic level, possible candidate templates to achieve these might be DNA miniarcs, which can stick due to base pairing, or functionalized fragments of cytoskeletal polymers such as actin and microtubules. The resulting self-assembled knots would have interesting mechanical and transport properties at the nanoscale, particularly if they could be made motile. At a more atomistic level, a natural choice is represented by helicates that have been recently used to design supramolecular constructs tied in trefoil and pentafoil torus knots. The abundance of the 8 19 knot among the helical self-assembled constructs (and for clusters of dipolar spheres too [19] ) suggests that it ought to be an ideal candidate for future attempts to design novel synthetic molecular knots. System setup In our simulations, we considered a collection of rigid helical templates with patchy ends. The body of each template was obtained by threading a portion of a helical centre line with touching hard spheres or beads with nominal diameter σ , see Fig. 1 . The template is next functionalized with two patchy interaction centres lying on the exposed surface of the terminal beads where it intersects the helical centre line, see Fig. 1 . The templates are treated as rigid bodies that interact with each other exclusively via the hard-core repulsion of the beads and the short-ranged attraction of the patches. A Weeks–Chandler–Andersen potential, that is, a shifted and truncated 12–6 Lennard–Jones potential, is used to enforce the excluded volume interaction of the hard spheres: where d ij is the distance between the i th and j th beads, ɛ is equal to the system thermal energy, k B T , and κ hs is an adimensional parameter quantifying how hard the potential is. Its value, together with that of the other parameters used, is given in the ‘Model parameters’ section. The repulsive interaction acts for distances and is zero otherwise. The pairwise attractive interaction of the patches has, instead, a Gaussian form: where κ patchy and σ patchy measure, respectively, the magnitude and range of the attractive interaction (again their values are given in the ‘Model parameters’ section). The dynamics of the i th hard-core bead, whose position vector we call r i , is described by a Langevin equation where m and γ are the mass and friction of the i th hard-core bead, the index j runs over the other hard-core beads, and ∇ i is the gradient operator with respect to the i th bead coordinates. The noise η is uncorrelated across the various beads and, for each of them, satisfies the usual fluctuation–dissipation conditions, 〈 η α ( t )〉=0 and 〈 η α ( t ) η β ( t ′)〉=2 k B Tγδ α, β δ t,t′ , with α and β running over the three Cartesian components. Similarly, the evolution of the k -th attractive patch is described by with the index l running over the other patchy centres. Notice that there is no interaction between the hard-core beads and the patchy centres because the latter exactly lie on the surface of the hard-core beads. The Langevin equations of motion for all beads are integrated numerically with the LAMMPS simulation package [44] with the rigid body constraint applied to each construct. The integration time step is Δ t =0.012 τ LJ , where and with m / γ =2 τ LJ as in ref. 45 . With these parameters, the templates’ typical Brownian time, that is, the time required by an isolated construct to diffuse over a distance equal to its radius of gyration, is τ B ∼ 40 τ LJ , see Fig. 6 . 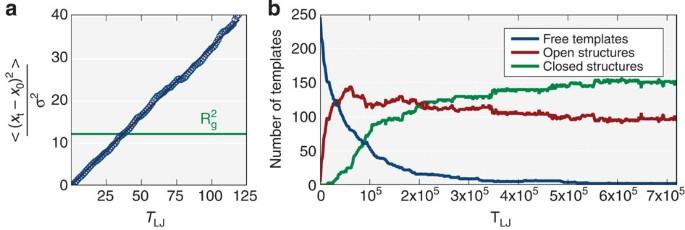Figure 6: Free dynamics and assembly kinetics of helical templates. (a) Time dependence of the mean square displacement of the centre of mass of a single template of geometryα=1.7πandh=1.0. It is seen that the time required to diffuse over a distance equal to its radius of gyration, that is, the characteristic Brownian time, is about equal to 40τLJ. (b) Typical time evolution of the number of templates that are unbound (blue curve) or bound in open (red) or closed (green) oligomers. The time evolution pertains to a single Langevin trajectory where 250 templates, of geometry (α=1.7π,h=1.0) are initially randomly arranged in the simulation box (hence they are all unbound). Stationarity ensues after about 2.5 × 105τLJ. The behaviour shown in both panels is typical of other template geometries too. Figure 6: Free dynamics and assembly kinetics of helical templates. ( a ) Time dependence of the mean square displacement of the centre of mass of a single template of geometry α =1.7 π and h =1.0. It is seen that the time required to diffuse over a distance equal to its radius of gyration, that is, the characteristic Brownian time, is about equal to 40 τ LJ . ( b ) Typical time evolution of the number of templates that are unbound (blue curve) or bound in open (red) or closed (green) oligomers. The time evolution pertains to a single Langevin trajectory where 250 templates, of geometry ( α =1.7 π , h =1.0) are initially randomly arranged in the simulation box (hence they are all unbound). Stationarity ensues after about 2.5 × 10 5 τ LJ . The behaviour shown in both panels is typical of other template geometries too. Full size image Model parameters The parameters of the attractive potential were set equal to κ patchy =25 and σ patchy =0.1 σ , while for the hard-core interactions we use κ hs =150. These parameters were chosen after several trials, and were adopted because it was found a posteriori that they satisfy a number of physics-based desiderata . In particular, the attractive potential is sufficiently short ranged that it avoids simultaneous binding of more than two patches that would, in turn, result in the formation of branched multimeric complexes. At the same time, the depth of the well is sufficient to guarantee that the unbinding time of two isolated templates is much larger than the characteristic microscopic time, τ B . Simulation details Each simulation includes 250 templates in a cubic box of volume with periodic boundaries. The desired total density of spheres in the simulation, ρ , is fixed by setting l b =( n m / ρ ) 1/3 , where n m is the number of hard spheres in the simulation box and ρ is set to 7.5 × 10 −3 σ −3 , corresponding to a volume fraction of ∼ 0.56% (other densities are considered in Fig. 4 ). Because the spherical particles are not individually dispersed in solution but are grouped to line the helical fragments, this volume fraction corresponds to an appreciable crowding of the templates. In fact, since each template typically consists of 15 beads, one has that its specific volume is about 2,000 σ 3 . The associated characteristic length scale, which measures the separation of neighbouring templates, is therefore ∼ 13 σ , which is comparable to the templates’ typical size (gyration diameter) which is ∼ 7 σ . The phase space was discretized with a triangular grid with α and h spacings, respectively, equal to 0.1 π and 0.1. The total number of sampled points is equal to 179. For each point considered in the ( α , h ) space, 20 independent starting configurations were randomly generated. For each simulation, the dynamical evolution was followed for a time span of at least 6,600 τ B , which suffices a posteriori to observe the stationarity plateau for the closure and knotting probability, see Fig. 6 . For each point in the ( α , h ) space, the system dynamics was thus followed, over various trajectories, for a total duration of at least 1.3 × 10 5 τ B and the closure and knotting probabilities were obtained by cumulating the data of the last snapshot of the 20 independent simulations. The density plot of Fig. 2 were obtained using a bicubic spline interpolation of the sampled data. The topological phase diagram of Fig. 3c is a Voronoi tasselation of phase space based on the dominant knot type (including the unknot) in each sampled point. Topological profiling The topological state of a ring is established from the crossings in one of its planar projections, specifically, from the succession of over- and under-passes. These are used to compute the Alexander determinants and, if needed, the Dowker codes [46] . The Alexander determinants are standard topological invariants that suffice to pinpoint the topological state of prime knots with fewer than 10 crossings in their minimal projection. More complex or composite knots are identified through the algebraic Dowker code, for which there exist lookup tables of all prime knotted components of up to 16 crossings. We used the tables made available in the Knotscape software package developed by M. Thistletwaite ( http://www.math.utk.edu/~morwen/knotscape ). How to cite this article: Polles, G. et al . Self-assembling knots of controlled topology by designing the geometry of patchy templates. Nat. Commun . 6:6423 doi: 10.1038/ncomms7423 (2015).